Perpendicular exchange bias in ferrimagnetic spin valves The exchange bias effect refers to the shift of the hysteresis loop of a ferromagnet in direct contact to an antiferromagnet. For applications in spintronics a robust and tunable exchange bias is required. Here we show experimental evidence for a perpendicular exchange bias in a prototypical ferrimagnetic spin valve consisting of DyCo 5 /Ta/Fe 76 Gd 24 , where the DyCo 5 alloy has the role of a hard ferrimagnet and Fe 76 Gd 24 is a soft ferrimagnet. Taking advantage of the tunability of the exchange coupling between the ferrimagnetic layers by means of thickness variation of an interlayer spacer, we demonstrate that perpendicular unidirectional anisotropy can be induced with desirable absolute values at room temperature, without making use of a field-cooling procedure. Moreover, the shift of the hysteresis loop can be reversed with relatively low magnetic fields of several hundred Oersteds. This flexibility in controlling a robust perpendicular exchange bias at room temperature may be of crucial importance for applications. After the discovery of the giant magnetoresistance [1] , [2] , the exchange bias (EB) effect has become an integral part of spintronics with implications for basic research and for numerous device applications like random access magnetic storage units and spin valves. Although its observation has been made only 60 years ago by Meiklejohn and Bean [3] when studying Co particles embedded in their natural oxide (CoO) matrix, the first EB system was engineered by nature long before, a few billion years ago, in grains of titanohaematite [4] . The origin of the EB effect is related to the magnetic coupling across the common interface shared by a ferromagnetic (FM) and an antiferromagnetic (AF) layer, when the system is cooled through the Néel temperature of the AF layer. The magnetic properties of the AF layer and the interface are crucial for understanding the magnetic properties of the EB systems [5] . Yet, these two magnetic components are difficult to access experimentally with laboratory tools because of a virtually vanishing magnetization of AF layers and a small volume of the magnetic interface. Important progress has been made by involving neutron and X-ray techniques to study the bulk part of the pinning layer and the interfacial magnetism [6] , [7] , [8] , [9] , [10] , [11] , [12] , [13] . For instance, in an archetypal CoO/FM bilayer, neutron scattering has revealed the origin of reduced EB. It was shown to be related to the anisotropic domain state of the AF system [12] . Using soft X-ray techniques, the frozen and rotatable spins [12] , [14] , [15] were observed in several systems, leading to a deeper understanding of the enhanced coercivity and the origin of the EB for systems with uncompensated AF interfaces. Larger efforts were dedicated to the understanding of the FM/AF EB systems with in-plane anisotropy of the ferromagnet [16] . Notably, Mangin and colleagues [17] , [18] , [19] , [20] have performed significant work on GdFe/TbFe ferrimagnetic soft/hard bilayers with in-plane anisotropy in which EB effects occur. EB was also studied in all coupled FM films with in-plane magnetized ferromagnets acting as pinning layers [21] , [22] . However, for applications, perpendicular uniaxial and unidirectional anisotropies are more desirable owing to a larger thermal stability of encoded information [23] . For instance, antiferromagnets in contact to ferromagnets with perpendicular anisotropy like Co/Pt multilayers and CoPt 3 layers have been shown to exhibit EB and all other macroscopic behaviour of EB systems, like training effect, enhanced coercivity and blocking temperature for the onset of the EB [23] , [24] , [25] , [26] . More recently, the perpendicular EB (PEB) was demonstrated in a novel exchange-coupled system Sm 1−0.028 Gd 0.028 Al 2 /SmAl 2 based on the zero magnetization ferromagnet Sm 1−0.028 Gd 0.028 Al 2 as the pinning layer [27] . The latter exhibits a compensation temperature where the antiparallel oriented spin and orbital moments cancel one another leading to a vanishing macroscopic magnetization of the ferromagnet [28] . In nearly all cases, the PEB is set through field-cooling or by in situ field growth procedures, similar to the AF/FM systems with in-plane anisotropy. In this article, we demonstrate that PEB can be set, controlled and reversed at room temperature in exchange-coupled ferrimagnetic systems, by making use of an interlayer exchange decoupling mechanism. As a prototype system, we have chosen artificial DyCo 5 /Ta(x)/Fe 76 Gd 24 spin-valve (SV) trilayers, where the hard ferrimagnet (HFi) DyCo 5 serves as a single magnetic domain pinning layer. In bulk form [29] and in thin films [30] , it has a magnetization compensation temperature and a spin reorientation temperature. As the orbital moment of Dy is nearly as large as the spin moment [31] , it is expected that DyCo 5 exhibits a large perpendicular anisotropy [32] , which qualifies it as a robust pinning layer. Owing to the vanishing orbital moment of Gd, the perpendicular magnetic anisotropy of Fe 76 Gd 24 (FeGd) is weak. Therefore, it acts as a soft ferrimagnetic layer (SFi). To induce a perpendicular unidirectional anisotropy, in a first step the soft and the hard ferrimagnets are partially decoupled by a Ta interlayer spacer, and in a second step hysteresis loops are measured, reversing the SFi magnetization while keeping the HFi magnetically saturated. In this way, the PEB can be set and even reversed without involving a field-cooling procedure. Perpendicular anisotropy with ferrimagnetic pinning layer The origin of EB in FM/AF and X/HFi (with X =FM or SFi) bilayers is related to the coupling across the interface shared by two adjacent magnetic layers. The magnetic state of the pinning layer interface has a crucial role in establishing a robust EB [5] . We exemplify below that, as a prerequisite for the occurrence of a strong PEB, the magnetic state of the interface of HFi pinning layer must be compensated. This contrasts the case of an AF pinning layer, where the magnetic state of the interface has to be uncompensated to establish a finite EB [5] . When the AF surface is fully uncompensated, one expects the largest EB to occur. In the opposite case, when the AF interface is fully compensated, the EB is expected to be zero [33] . The last situation is depicted in Fig. 1a . The magnetic moments in the AF layers are coupled antiferromagnetically. Across the interface, the coupling between neighbouring spins is assumed to be ferromagnetic. One can analyse the impact of this compensated magnetic state on the EB in terms of interfacial energy. The interfacial energy is calculated as E kl =− J i S k S l per pair of nearest neighbour spins at the interface [33] . Then, the EB field is proportional to 2* σ / A , where σ is the available energy and A is the unit area [33] . One observes in Fig. 1a that the first and the third (from the left) spin pair exhibits a parallel orientation; therefore they contribute negatively to the interface energy. However, the second and the fourth spin pairs contribute positively to the interface energy because the spins in the AF are oppositely oriented with respect to the FM spin. As a result, the interfacial energy vanishes for a compensated AF interface leading to a forbidden EB effect. 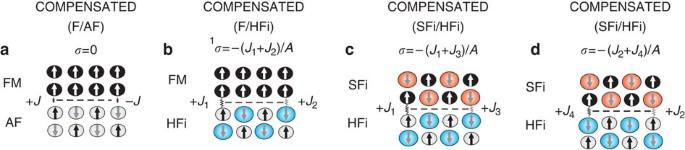Figure 1: Perpendicular unidirectional anisotropy with ferrimagnets. (a) Schematic view of a compensated AF interface. The interfacial energy is zero for this configuration, therefore no EB is allowed to occur. (b–d) A schematic view of a compensated hard ferrimagnetic interface in contact to a ferromagnet and a soft ferrimagnet, respectively. The larger circle designates the RE metal atom and the smaller one designates the TM atom. This interface does not exhibit frustrated bonds, leading to a maximum interfacial energyσfor EB to occur. The difference between (c) and (d) is the relative offset between the layers by one site. Figure 1: Perpendicular unidirectional anisotropy with ferrimagnets. ( a ) Schematic view of a compensated AF interface. The interfacial energy is zero for this configuration, therefore no EB is allowed to occur. ( b – d ) A schematic view of a compensated hard ferrimagnetic interface in contact to a ferromagnet and a soft ferrimagnet, respectively. The larger circle designates the RE metal atom and the smaller one designates the TM atom. This interface does not exhibit frustrated bonds, leading to a maximum interfacial energy σ for EB to occur. The difference between ( c ) and ( d ) is the relative offset between the layers by one site. Full size image An opposite situation occurs for bilayers with ferrimagnetic pinning layers. This is depicted in Fig. 1b–d . For the sake of simplicity, we consider the HFi layer to be magnetically compensated. For instance, this can be achieved at the magnetization compensation temperature, where the magnetizations of the two sublattices are equal, leading to a vanishing total magnetization, just as in antiferromagnets. In Fig. 1b , the HFi layer is coupled to a FM layer. For this compensated HFi interface, the interfacial energy does not vanish. The first and third spin pairs contribute negatively to the total energy. The coupling between the transition metal and the rare-earth metal is AF across the interface (and within the HFi layer). Therefore, the second and the fourth spin pairs contribute also negatively to the interfacial energy. As a result, a compensated interface of a HFi layer leads to a maximum EB. When the pinned layer is a SFi, a similar situation occurs as shown in Fig. 1c,d . All the spin pairs contribute negatively to the interface; therefore the compensated nature of HFi leads to maximum interfacial energy for both FM and SFi pinned layers. The occurrence of a highest available interfacial energy for a compensated interface of a HFi layer does not necessarily lead to a shift of the hysteresis loop for the pinned layer. A critical condition has to be obeyed for the EB to occur [5] , namely Kt / J >1, where K is the HFi anisotropy, t is the thickness of the HFi layer and J is the interfacial coupling constant. Therefore, when the coupling is large, the above condition prevents the EB to occur. Our approach here is to make use of an interlayer spacer for tuning down the coupling strength to values that fulfills the critical condition for EB. Magnetic properties of the ferrimagnetic films The magnetic properties of the individual HFi and SFi ferrimagnetic layers prepared as separate samples were studied by soft X-ray magnetic circular dichroism (XMCD). In Fig. 2a , we show the temperature dependence of the coercive field and the normalized remanent magnetization for the single DyCo 5 (250 Å) layer. These data have been extracted from the hysteresis loop measurements at the L 3 resonant energy of Co. The DyCo 5 layer exhibits two magnetic transition temperatures, a magnetization compensation temperature and a spin reorientation temperature. The magnetization compensation temperature occurs at about T comp =120 K where the sum of the orbital and spin moments of the Co layer equals the magnetic moment of Dy, leading to a vanishing net magnetization of the film. For systems with uniaxial magnetic anisotropy, the coercive field is proportional to the magnetic anisotropy of the film and inversely proportional to the total magnetization [5] . Therefore, at the magnetization compensation temperature, the coercive field diverges as the net magnetization approaches towards zero, as shown in Fig. 2a . The compensation temperature can also be identified by the inverted hysteresis loop below T comp as compared with the one measured above T comp as shown in the insets of Fig. 2a . Below T comp , the Dy magnetic moment becomes dominant and therefore the Co moment is oriented antiparallel with respect to the applied magnetic field. Above T comp , the magnetic moment of Co is larger than the one of Dy and therefore, it is oriented parallel to the external field. At higher temperatures, the DyCo 5 film exhibits a spin reorientation temperature ( T R =350 K). We observe that the uniaxial magnetic anisotropy rotates from out-of-plane, below T R to in-plane, above T R as clearly verified by the different shapes of the hysteresis loops in both regions shown in the insets of Fig. 2a . Below T R , the hysteresis loops of the DyCo 5 remain squared as exemplified in the inset of Fig. 2a , and exhibit high remanent magnetization equal to the saturation magnetization. These square loops with their high remanence at room temperature are nearly ideal properties of films with uniaxial perpendicular anisotropy. The hysteresis loop above T R has a very low remanent magnetization, and is characteristic for a hysteresis loop measured along the hard axis of a thin magnetic film with uniaxial anisotropy. 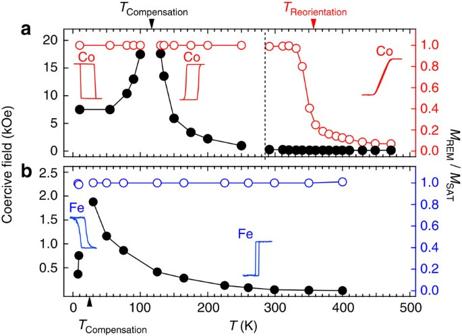Figure 2: Ferrimagnetic properties of the individual films. (a) The temperature dependence of the coercive field (filled black circles) and the remanent magnetization (open red circles) extracted from hysteresis loops measured for a 250-Å-thick DyCo5sample. The magnetization compensation temperature (Tcomml_mpDyCo5=120 K) is clearly visible at the temperature where the coercive field diverges, whereas the reorientation temperature (TRDyCo5=350 K) is distinguishable as a change of the remanent magnetization. The insets show hysteresis loops belowTcomp, betweenTcompandTR, and aboveTR. (b) The temperature dependence of the coercive field (filled black circles) and the normalized remanent magnetization (open blue circles) for the FeGd film extracted from the hysteresis loops. In the inset are two representative hysteresis loops measured below and well above the compensation temperature (TcompFeGd=14 K). The external magnetic field was applied perpendicular to the sample surface. Figure 2: Ferrimagnetic properties of the individual films. ( a ) The temperature dependence of the coercive field (filled black circles) and the remanent magnetization (open red circles) extracted from hysteresis loops measured for a 250-Å-thick DyCo 5 sample. The magnetization compensation temperature ( T comml_mp DyCo 5 =120 K) is clearly visible at the temperature where the coercive field diverges, whereas the reorientation temperature ( T R DyCo5 =350 K) is distinguishable as a change of the remanent magnetization. The insets show hysteresis loops below T comp , between T comp and T R , and above T R . ( b ) The temperature dependence of the coercive field (filled black circles) and the normalized remanent magnetization (open blue circles) for the FeGd film extracted from the hysteresis loops. In the inset are two representative hysteresis loops measured below and well above the compensation temperature ( T comp FeGd =14 K). The external magnetic field was applied perpendicular to the sample surface. Full size image It is essential that the SFi exhibits a low coercive field and a high magnetic remanence characteristic for a well-defined perpendicular uniaxial anisotropy. These magnetic properties of the SFi layer were tuned by means of stoichiometry variation. The characterization of a single Fe 76 Gd 24 (500 Å) layer that fulfils the required magnetic behaviour is shown in Fig. 2b . The hysteresis loops were measured at the L 3 resonant energy of Fe. The compensation temperature of the FeGd film was tuned [34] to lower temperatures in order to obtain a square hysteresis loop with a high remanent magnetization at room temperature. This ideal squareness with a low coercive field of about 60 Oe as well as the compensation nature of the FeGd alloy are clearly demonstrated in the insets of Fig. 2b . Decoupling the ferrimagnetic layers When the SFi (FeGd) and the HFi (DyCo 5 ) layers are set in direct contact, the exchange coupling between them is so strong that the magnetization of the SFi layer follows the one of the HFi layer. Therefore, in order to observe PEB, it is essential to partially decouple the ferrimagnetic layers as presented further on. In Fig. 3 , we show the hysteresis loops of the Si 3 N 4 /Ta(50 Å)/DyCo 5 (250 Å)/Ta(x Å)/FeGd(500 Å) trilayers for several Ta thicknesses. The 50 Å Ta layer next to the Si 3 N 4 substrate serves as an adhesion layer and has no role in our further discussion. When the FeGd and DyCo 5 films are in direct contact, the coercive field is the same for both layers, H c =350 Oe as observed in Fig. 3a . Fe and Co are aligned parallel to the field and exhibit a parallel interfacial exchange coupling. Dy and Gd magnetic moments are also parallel exchange coupled but antiparallel oriented with respect to the external field. This is the most favourable configuration leading to a strong coupling between these layers. The other situation, when measuring in between the compensation temperatures of the two ferrimagnets, would lead to frustrated magnetic moments at the interface because of competing interactions between a rare earth dominated ferrimagnet and a transition metal dominated one. In order to allow EB to occur, one needs to partially decouple these two layers. This is achieved by introducing a Ta interlayer of suitable thickness. We observe that for 1, 2 and 3 Å thick Ta interlayer, the DyCo 5 and FeGd films are still reversing together as shown in Fig. 3b . A sizeable decoupling appears only when Ta is about 5 Å thick ( Fig. 3c ). When the Ta thickness is further increased to 10 Å, the interlayer exchange coupling strength diminishes and therefore the coercive field of the FeGd layer further decreases ( Fig. 3d ). For fully decoupled layers, the coercive field of the SFi layer is H c =60 Oe ( Fig. 3e ). Note that the coercive field of the DyCo 5 layer does not vary considerably as a function of the spacer layer thickness, which is in strong contrast with the large variation of the coercive field of the FeGd layer. This further confirms the hard and soft nature of the magnetic properties of these two films, in agreement with their much different values for the orbital moments. Given that the total magnetizations of the SFi and HFi layers do have finite values at room temperature, a SV configuration can be induced for the partially decoupled trilayers. Reversing the net magnetization of FeGd in a saturated state of DyCo 5 layer leads to an antiparallel orientation of the net magnetizations of both ferrimagnetic films, just like in classical FM SV systems [35] . One conceptual difference between our perpendicular ferrimagnetic SV and the FM SV systems is that the interlayer is used here to decouple only partially the ferrimagnetic layers, while for the classical case (AF/FM/spacer/FM) an interlayer spacer is used to fully decouple the FM-free layer from the FM pinned layer. 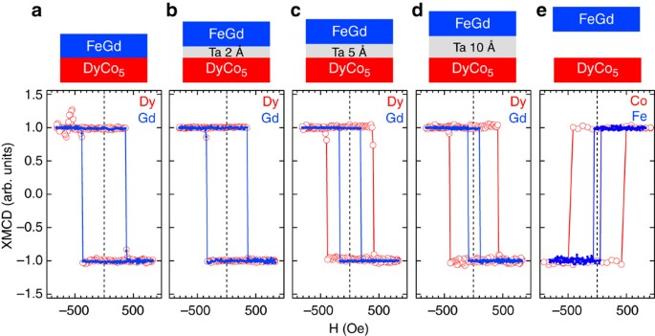Figure 3: Element specific XMCD hysteresis loops measured for samples with different interlayer Ta thicknesses. For a Ta thickness of 0 Å (a) and 2 Å (b), both ferrimagnetic layers reverse together. For 5 Å (c) and 10 Å (d) Ta thicknesses, the magnetizations of FeGd and DyCo5are partially decoupled. The hysteresis loops of individual layers are shown in (e). The measurements were performed at room temperature. The statistical errors are smaller than the symbol size. Figure 3: Element specific XMCD hysteresis loops measured for samples with different interlayer Ta thicknesses. For a Ta thickness of 0 Å ( a ) and 2 Å ( b ), both ferrimagnetic layers reverse together. For 5 Å ( c ) and 10 Å ( d ) Ta thicknesses, the magnetizations of FeGd and DyCo 5 are partially decoupled. The hysteresis loops of individual layers are shown in ( e ). The measurements were performed at room temperature. The statistical errors are smaller than the symbol size. Full size image Room temperature control of PEB Taking advantage of the partial decoupling of the FeGd and DyCo 5 , we demonstrate in Fig. 4 that the hysteresis loops of FeGd can be shifted and the shift's sign even reversed without involving a field-cooling procedure. In the left column, we show the measured data corresponding to the sample with a Ta interlayer thickness of 5 Å. When the hysteresis loop is measured between −900 Oe to +900 Oe and backwards, both element-specific hysteresis loops of the DyCo 5 and FeGd layers are centred with respect to the external field as shown in Fig. 4a . However, after saturating the system in a positive field higher than the coercive field of HFi and measuring the hysteresis loop of the FeGd layer from 300 to −300 Oe and backwards, a shift of the hysteresis loop occurs ( Fig. 4b ), revealing the presence of a unidirectional anisotropy. The EB and the coercive fields are H EB =−80 Oe and H c =112 Oe, respectively. Note that the coercive field of the biased FeGd is higher than the coercive field when unbiased, as expected (compare Fig. 4b with Fig. 3e ). Please also note that the hysteresis loops in Fig. 4a , although centred with respect to the field axis, are not unbiased. They are centred because we reverse the unidirectional anisotropy by reversing the DyCo 5 layer during the field cycle. As a result, the EB field adds to the coercivity in the Fig. 4a . For the scenario in Fig. 4b , the DyCo 5 film remains saturated in a single magnetic domain state, and through interlayer exchange coupling a unidirectional anisotropy is mediated in the FeGd layer, according to the coupling mechanism described at the beginning of this section. When the system is saturated in a negative field smaller than the coercive field of the HFi layer and a subsequent hysteresis loop is measured from −300 to +300 Oe and backwards, the magnetization curve of FeGd is shifted to the opposite side, as shown in Fig. 4c . This demonstrates that the unidirectional anisotropy can be reversed in relatively low fields and without involving any field-cooling procedure. The single magnetic domain state of the pinning layer is of crucial importance also for the stability of the EB field. In Supplementary Fig. S1 , we show that the coercive and EB fields remain stable as a function of the loop index, demonstrating that a training effect is essentially absent. A magnetic multi-domain state in the pinning layer not only diminishes drastically the absolute value of the EB field but it also mediates a strong EB reduction upon consecutive cycling (training effect) [12] , [21] . 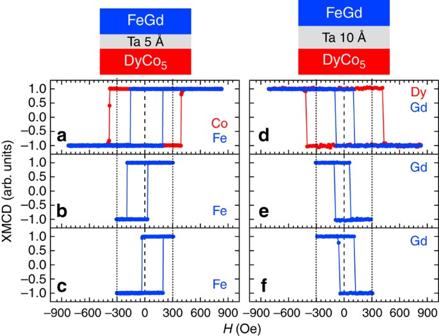Figure 4: Exchange-biased hysteresis loops for two representative samples. Left column: (a–c) the hysteresis loops measured for a sample with a 5 Å Ta interlayer spacer. Panel (a): the hysteresis loops of the DyCo5and FeGd films were measured from 900 to −900 Oe. Panel (b): the system was saturated in a positive field of +3,000 Oe and consecutively a hysteresis loop was measured between +300 Oe and −300 Oe. Panel (c): the system was saturated in a negative field of −3,000 Oe and consecutively a hysteresis loop was measured between −300 Oe and +300 Oe. Right column: (d–f) the same scenario was followed for a sample with a Ta interlayer thickness of 10 Å. The dotted vertical lines mark the +300 Oe and −300 Oe fields. The statistical errors are smaller than the symbol size. Figure 4: Exchange-biased hysteresis loops for two representative samples. Left column: ( a–c ) the hysteresis loops measured for a sample with a 5 Å Ta interlayer spacer. Panel ( a ): the hysteresis loops of the DyCo 5 and FeGd films were measured from 900 to −900 Oe. Panel ( b ): the system was saturated in a positive field of +3,000 Oe and consecutively a hysteresis loop was measured between +300 Oe and −300 Oe. Panel ( c ): the system was saturated in a negative field of −3,000 Oe and consecutively a hysteresis loop was measured between −300 Oe and +300 Oe. Right column: ( d–f ) the same scenario was followed for a sample with a Ta interlayer thickness of 10 Å. The dotted vertical lines mark the +300 Oe and −300 Oe fields. The statistical errors are smaller than the symbol size. Full size image To further demonstrate that the absolute value of the PEB field can also be controlled, we show in the right column of Fig. 4 the magnetization for a sample with 10 Å Ta interlayer thickness. The same procedure (as for the sample with 5 Å Ta) was applied to reveal the occurrence of the unidirectional anisotropy in FeGd. The characteristic hysteresis loops shown here are measured by probing the rare earth elements (at the M 5 resonant energy), which demonstrates also their intrinsic AF orientation with respect to the transition metal. The coercive field and the EB for the SFi layer are clearly smaller as compared with the sample with thinner Ta thickness. Therefore, by varying the interlayer thickness one can tune in a controlled manner the absolute value of the EB and coercive fields. The coupling mechanism with HFi pinning layers is fundamentally different as compared with the established mechanism of EB with AF pinning layers. While for the latter one it is required that the AF exhibits a magnetically uncompensated interface for EB to be established, in the former case a compensated HFi interface is required for the largest EB effect to occur. Moreover, for FM/AF EB systems with in-plane anisotropy, the thickness of the interlayer does not exhibit a cutoff behaviour. Submonolayer dusting of the interface is sufficient to dramatically reduce the absolute values of the EB and coercive fields [36] . This is different for our system, where a much larger thickness of Ta, equal to 5 Å, was needed to allow EB to occur. The critical thickness for the interlayer can be understood based on models for EB [5] . For instance, in AF/FM bilayers, the onset of EB occurs for a critical AF thickness, which is given by the condition R =( K AF t AF )/ J EB ≥1, where the K AF and t AF are the anisotropy and the thickness of the AF, respectively, and J EB is the interfacial coupling constant. This implies that the AF thickness needs to be increased until the AF layer can resist the interfacial torque that acts during the rotation of the ferromagnet [15] . In our case, the thickness and the anisotropy of the HFi layer are held constant; therefore the interfacial coupling has to be decreased by increasing the thickness of the interlayer until the condition above is satisfied. The dipolar coupling between the macroscopic magnetization of the two ferrimagnetic layers also has a role, contributing, however, minimally to the absolute critical thickness of the interlayer. In fact, the enhanced coercive fields of the SFi hysteresis loops in Fig. 4 can be partially attributed to dipolar coupling. For instance, when the FeGd magnetization reverses first, the net magnetizations of the HFi and SFi layers are in an unfavourable antiparallel situation, therefore an enhanced coercive field is observed. This is different with respect to the EB with in-plane anisotropy where the stray fields are not present leading to a vanishing dipolar coupling. In conclusion, we have demonstrated that PEB in ferrimagnetic DyCo 5 /Ta(x)/Fe 76 Gd 24 alloys, where the DyCo 5 layer has the role of a single magnetic domain hard ferrimagnet and the FeGd alloy acts as a soft ferrimagnet, can be controlled in a flexible and robust manner. Taking advantage of the tunability of the interlayer exchange coupling, we have shown that PEB can be induced without making use of a field-cooling procedure. This was achieved by carefully engineering the magnetic properties of the soft ferrimagnet and the thickness of the partially decoupling interlayer. Owing to the strong coupling between the DyCo 5 and FeGd, the EB occurs above a critical thickness of Ta interlayer, at 5 Å. The absolute value of the EB can be tuned through the thickness of the interlayer spacer and even reversed with relatively low magnetic fields of several hundred Oersteds. This flexibility in controlling a robust PEB at room temperature may be of outmost importance for applications in modern ultrafast storage media [37] . Sample preparation The samples were grown by magnetron sputtering (MAGSSY chamber at HZB) in an ultraclean Argon atmosphere of 1.5×10 −3 mbar with a base pressure of <5×10 −9 mbar at the deposition temperature of 300 K. The stoichiometry of the ferrimagnetic alloys was controlled by varying the deposition rate of separate chemical elements in a co-evaporation scheme. As substrates, we used Si 3 N 4 membranes. XMCD from ferrimagnetic films XMCD was measured in a transmission geometry [38] , [39] at BESSY II using the ALICE diffractometer [40] installed at the PM3 bending magnet beamline. The study of the DyCo 5 layer in high fields was performed with the high-field endstation at the beamline UE46-PGM1 installed at the electron storage ring BESSY II. The measurements were performed by detecting the external field-dependent transmitted intensity of the circularly polarized soft X-rays with the energy set to the experimental L 3 resonant edges of Co(780.4 eV) and Fe(709.4 eV), and M 5 resonant edges of Gd(1,187 eV) and Dy(1,297 eV). Circularly polarized soft X-rays are impinging at normal incidence on the sample placed in an external magnetic field set parallel to the beam direction. The transmitted intensity is measured by a Si photodiode, which is insensitive to applied magnetic fields. Typical experimental spectra for a DyCo 5 /Ta/FeGd sample are shown in Fig. 5b–e . By varying the energy of the circularly polarized light and measuring the normalized transmitted intensity for two opposite saturating fields, one observes a strong variation of intensity at the absorption edges. The experimental XMCD curves are then extracted as the logarithm of the ratio of the transmitted intensities for positive and negative field, respectively. Inspecting the polarity of the XMCD signal at the absorption edges, one obtains information about the relative orientation of the sublattice magnetization components. For instance, the XMCD at the Co L 3 edge is negative whereas the XMCD at the M 5 edge of Dy is positive. This shows that the magnetic moments of Co and Dy are oriented antiparallel with respect to each other. Similarly, the XMCD signals at the L 3 edge of Fe and at the M 5 edge of Gd have opposite signs, demonstrating the ferrimagnetic nature of the layers. Most important, for the case of interfacial (or interlayer) coupled films, the coupling sign between the magnetic moments of adjacent magnetic layers can be directly extracted owing to the element-specific sensitivity of the XMCD technique. In our case, the transition metal (Fe and Co) are oriented parallel with respect to each other and the rare earth metals (Gd and Dy) are also parallel oriented. 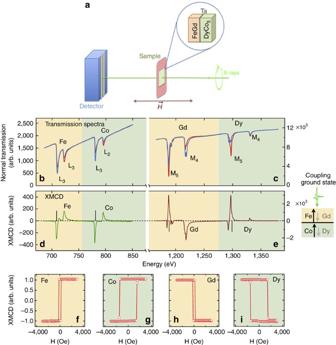Figure 5: XMCD from ferrimagnets. (a) Sketch of the transmission geometry with circularly polarized soft X-rays. The normalized transmitted spectra are shown in (b,c), measured for opposite orientations of the magnetic field (±3 kOe). In (d) and (e) the experimental XMCD spectra are shown. By fixing the photon energy at specific absorption edges and measuring the transmitted intensity while sweeping the external magnetic field, one obtains the element-specific hysteresis loops. Typical hysteresis loops measured at the L3absorption edges of Fe and Co, and M5absorption edges of Dy and Gd are shown in (f) and (g), and (h) and (i), respectively. The measurements have been performed for a DyCo5/Ta(5 Å)/FeGd sample at a temperature of 250 K, which is well above the compensation temperatures for both DyCo5and FeGd layers. Figure 5: XMCD from ferrimagnets. ( a ) Sketch of the transmission geometry with circularly polarized soft X-rays. The normalized transmitted spectra are shown in ( b , c ), measured for opposite orientations of the magnetic field (±3 kOe). In ( d ) and ( e ) the experimental XMCD spectra are shown. By fixing the photon energy at specific absorption edges and measuring the transmitted intensity while sweeping the external magnetic field, one obtains the element-specific hysteresis loops. Typical hysteresis loops measured at the L 3 absorption edges of Fe and Co, and M 5 absorption edges of Dy and Gd are shown in ( f ) and ( g ), and ( h ) and ( i ), respectively. The measurements have been performed for a DyCo 5 /Ta(5 Å)/FeGd sample at a temperature of 250 K, which is well above the compensation temperatures for both DyCo 5 and FeGd layers. Full size image The element-specific hysteresis loops are recorded by setting the photon energy to the experimental L 3 absorption edges of the transition metal or to the M 5 absorption edges of the rare earth and measuring the transmitted intensity while sweeping the magnetic field. Typical hysteresis loops obtained for Co, Dy, Fe and Gd are shown in Fig. 5f–i . The polarity of the hysteresis loops reflects also the relative orientation of the elemental magnetic moments. Additionally, it provides intrinsic magnetic parameters, that is, the coercive and EB fields for each probed element. In this way, element-specific hysteresis loops can be used to probe the complex magnetic behaviour of exchange-coupled films, demonstrating also the coupling ground state of these layers. How to cite this article: Radu, F. et al . Perpendicular exchange bias in ferrimagnetic spin valves. Nat. Commun. 3:715 doi: 10.1038/ncomms1728 (2012).